X-ray photonic microsystems for the manipulation of synchrotron light Photonic microsystems played an essential role in the development of integrated photonic devices, thanks to their unique spatiotemporal control and spectral shaping capabilities. Similar capabilities to markedly control and manipulate X-ray radiation are highly desirable but practically impossible due to the massive size of the silicon single-crystal optics currently used. Here we show that micromechanical systems can be used as X-ray optics to create and preserve the spatial, temporal and spectral correlation of the X-rays. We demonstrate that, as X-ray reflective optics they can maintain the wavefront properties with nearly 100% reflectivity, and as a dynamic diffractive optics they can generate nanosecond time windows with over 100-kHz repetition rates. Since X-ray photonic microsystems can be easily incorporated into lab-based and next-generation synchrotron X-ray sources, they bring unprecedented design flexibility for future dynamic and miniature X-ray optics for focusing, wavefront manipulation, multicolour dispersion, and pulse slicing. Devices based on microelectromechanical systems (MEMS) when combined with micro-optics have found a wide range of photonics applications. These include high-resolution imaging and displays [1] , biomedical diagnostics and bioimaging [2] , [3] , and optical communications [4] , [5] , all of which rely on the ability of the device to control the temporal and spectral shape of light pulses. Most MEMS use silicon as the structural material that act as mirrors, gratings and lenses to perform device functions such as microfocusing, high-speed modulation, beam-splitting, spectral filtering, wavelength dispersion, waveguiding and scanning. We ask the question whether these photonic functions of MEMS can also be extended to the X-ray wavelength since they have as yet unexplored applications in X-ray telescopes [6] , clinical X-ray imaging facilities [7] , at current and future-generation X-ray sources [8] , [9] and in future compact X-ray sources based on the accelerator-on-a-chip concept [10] , [11] . Fortunately, the single-crystal silicon that is a preferred material for use in MEMS [12] is also the mainstay of reflective and diffractive X-ray optics for monochromatization, reflection, focusing and dispersion [13] , [14] . However, the X-ray applications use silicon single-crystals that are 2–5 orders of magnitude larger in size and 6–15 orders higher in mass compared with MEMS optics. If X-ray optics can be developed with size, weight and performance comparable to MEMS optics, they will enable new static and dynamic functions that are currently not possible. For example, one could perform ultrafast adaptive X-ray optical functions for biological and materials imaging [15] , and real-time X-ray spectroscopy with microsecond temporal resolution, which will allow the investigation of the dynamic processes responsible for the electronic, spin and structural functions in organic and inorganic materials [16] , [17] , [18] , [19] . When incorporated into existing X-ray synchrotron sources, MEMS-based X-ray optics could be used to implement compact non-accelerator approaches to control pulse characteristics such as shape and phase of an X-ray wavefront. In spite of the promise and potential of this technology, no studies have so far assessed the effectiveness of MEMS devices as X-ray optics [20] . Here we demonstrate the unique capabilities of the single-crystal Si MEMS-based X-ray optics to manipulate X-ray radiation. Using coupled electromagnetic and mechanical FEM (finite element modelling) simulations, we have designed MEMS devices that are operated in an unexplored oscillation frequency and amplitude regime suitable for X-ray optics. We implemented a dynamic diffracting element to generate nanosecond time windows with very high angular velocities at over 100-kHz repetition rates. Furthermore, from the discussion to follow, it becomes apparent that by utilizing MEMS technology for X-rays, a new generation of photonics microsystems for X-ray wavelengths will be possible in the near future. MEMS-based elements can be effective as an X-ray mirror only if the surface is atomically smooth and flat to efficiently reflect photons of Ångstrom wavelength at grazing incidence angles (without distorting) the X-ray wavefront. To reveal whether MEMS mirrors possess these properties, we designed and fabricated torsional MEMS devices with a single oscillating element of single-crystal Si (100) that is 10-μm thick and 500-μm × 500-μm in lateral dimension. It is suspended by a pair of torsional flexures, which are anchored to the substrate, as shown in the scanning electron microscopy image ( Fig. 1a ). The flexures allow the crystal to rotate in the torsional oscillation mode about an axis joining the anchors. The device is fabricated using a SOI (silicon-on-insulator) wafer that provides the single-crystal Si layer necessary to diffract X-rays. The substrate beneath the crystal is removed to allow large out-of-plane oscillations and to allow the transmission of X-rays. The excitation is provided by in-plane comb-drive actuators, which are inter-digitated capacitors that provide torque with high force density [1] , [21] (see Supplementary Data 1 and Supplementary Fig. 1 ). The static X-ray reflectivity of the mirror at grazing incidence was measured while the device is not energized. With a two-dimensional X-ray detector, the incident and reflected beams were recorded simultaneously, as shown in Fig. 1b while the device was rotated from zero to the critical angle of the Si mirror (0.18°). The reflected beam was shown to be in well-defined spots indicating that the X-rays reflect off a high-quality mirror surface. This is confirmed by a quantitative X-ray reflectivity scan ( Fig. 1c ), which demonstrates the reflection efficiency predicted by theory [14] . The measured reflectivity drops abruptly at the critical angle, again confirming a smooth and flat mirror surface. Therefore, the micromachined mirrors have comparable quality of conventional large X-ray mirrors and can be used to control the X-ray wavefront, for example, to optimally achieve X-ray focusing with an array of such elements and adaptive controls. 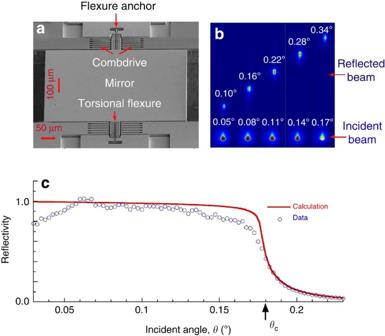Figure 1: Grazing incidence reflectivity of fabricated torsional MEMS device. (a) The scanning electron microscopy image of the 500-μm × 500-μm MEMS device shows the reflective crystal surface, the comb-drive actuators and torsional flexures. Note the perspective angle of the image is about 60° so that the square mirror appears to be rectangular. X-rays impinge on the surface of the mirror in the horizontal direction, perpendicular to the torsional flexures. (b) Both the reflected beam and incident beam are recorded on a CCD (charge-coupled device) camera. The reflected beam is a well-defined spot on the area detector indicating the X-rays are reflected from a high-quality smooth mirror surface. (c) A point detector measures the intensity of the reflected beam with respect to incidence angle and shows that reflection efficiency matches well with theory. The abrupt reflectivity drop at θc(≈0.18°) implies a high degree of flatness. Figure 1: Grazing incidence reflectivity of fabricated torsional MEMS device. ( a ) The scanning electron microscopy image of the 500-μm × 500-μm MEMS device shows the reflective crystal surface, the comb-drive actuators and torsional flexures. Note the perspective angle of the image is about 60° so that the square mirror appears to be rectangular. X-rays impinge on the surface of the mirror in the horizontal direction, perpendicular to the torsional flexures. ( b ) Both the reflected beam and incident beam are recorded on a CCD (charge-coupled device) camera. The reflected beam is a well-defined spot on the area detector indicating the X-rays are reflected from a high-quality smooth mirror surface. ( c ) A point detector measures the intensity of the reflected beam with respect to incidence angle and shows that reflection efficiency matches well with theory. The abrupt reflectivity drop at θ c (≈0.18°) implies a high degree of flatness. Full size image As an X-ray diffractive optics, the MEMS crystal element also needs to be strain-free over the X-ray penetration volume to achieve high diffraction efficiency at both static and dynamic conditions. The X-ray rocking curve of the MEMS optics ( Fig. 2a ) is measured with 8 keV X-rays around the Si(400) Bragg angle, θ B of 34.807°, using a high-resolution diffractometer (see Supplementary Methods and Supplementary Fig. 2 ). A typical rocking curve of the crystal is shown in Fig. 2b with a peak reflectivity close to 50%. It consists of a narrow and intense Si(400) peak and additional intensity in the broad peaks above θ B . These originate from the multiple lattice-strained surface-states due to shallow diffusive phosphorous dopant layers introduced on the crystal surface during the MEMS fabrication. Besides a Gaussian to fit the Si(400) peak, the intensity profile was numerically fitted with two Gaussian peaks centred at 0.0038° and 0.0091° above the Si(400) peak, which agrees with a comprehensive investigation of phosphorous doped Si [22] . The large angular separation of the shoulder peaks from the Si(400) peak and their lower intensity allowed an accurate analysis of the Si(400) peak. The Si(400) peak (red line in Fig. 2b ), also modelled as a Gaussian, has a full-width-at-half-maximum, Δ θ (400) of 0.0034° (59 microradians). The above-described 3-Gaussian analysis of the diffraction profile yields an extremely good fit to the measured data as shown in Fig. 2b . We would, however, emphasize that the dopant-induced strain present in this device is due to the fixed multi-user MEMS fabrication process [23] from the manufacturing foundry. The stress due to the dopant layer is now well understood and has not interfered with our effort to optimize other parameters of the MEMS mirrors for dynamic X-ray optics. The dopant effect can be eliminated in the future by using a custom foundry run. 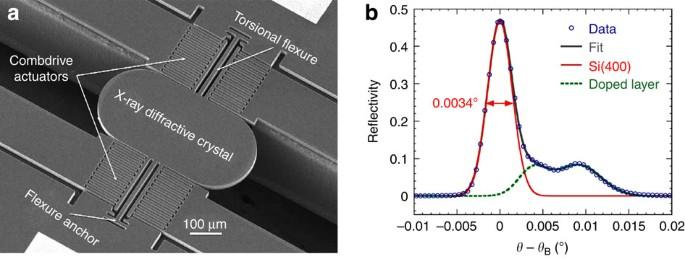Figure 2: X-ray static rocking curve of fabricated torsional 75-kHz MEMS device. (a) The scanning electron microscopy of 25-μm thick 75-kHz MEMS with rounded edges shows the diffractive crystal surface, the comb-drive actuators and torsional flexures. (b) The normalized static rocking curve measured at 8 keV shows a prominent Si(400) diffraction peak with nearly 50% reflectivity and broad peaks on the right, which originate from the lattice strain due to the dopant layer discussed in the text. Future fabrication will eliminate this dopant layer during the manufacturing process. Figure 2: X-ray static rocking curve of fabricated torsional 75-kHz MEMS device. ( a ) The scanning electron microscopy of 25-μm thick 75-kHz MEMS with rounded edges shows the diffractive crystal surface, the comb-drive actuators and torsional flexures. ( b ) The normalized static rocking curve measured at 8 keV shows a prominent Si(400) diffraction peak with nearly 50% reflectivity and broad peaks on the right, which originate from the lattice strain due to the dopant layer discussed in the text. Future fabrication will eliminate this dopant layer during the manufacturing process. Full size image In the case of diffraction of a monochromatic beam, if the crystal were strain and defect free, the value of Δ θ (400) would be determined by a convolution between the angular and energy widths of the incoming beam and the Darwin width of the Si(400) crystal (ref. 14 ), which was calculated to be 0.0028° (49 microradians). The measured Δ θ (400) is ∼ 20% broader, which can be accounted from the static deformation strain of the suspended 25-μm thick MEMS crystal. The static deformation of 0.0014° (24 microradians) was estimated from the measured concave curvature of the crystal from both optical metrology and X-ray data. With the static deformation accounted for, the predicated rocking curve width of 0.0032° (55microradians) is in good agreement with the measured value. The concept of using MEMS in the X-ray wavelength range as a dynamic diffractive optic for a monochromatic beam is shown schematically in Fig. 3a . A thin single-crystal Si MEMS can diffract or transmit X-ray radiation just by a change in its relative orientation to the incident X-ray beam. An oscillating MEMS device will diffract the X-rays over a short period of time when the Bragg condition is satisfied and it will transmit the X-rays over the rest of the cycle. This was demonstrated experimentally in Fig. 3b,c that show, respectively, the incident 6.518-MHz X-ray pulses from the APS storage ring and a diffracted X-ray pulse when an incident 100-ps X-ray pulse struck the Si MEMS and coincides with the Si(400) Bragg angle of the oscillating single crystal. The X-rays pulses were measured with a fast-response avalanche photodiode detector operating in a charge-integrating mode (see Supplementary Methods ). The MEMS angular speed determines the width of the diffractive time window over which the Bragg condition is fulfilled ( Fig. 3d ). Varying the delay between the X-ray pulse and the instance when the crystal sweeps through its Bragg angle can reveal the profile of the window in the time domain. To implement this concept successfully, a MEMS device has to perform as an X-ray diffractive element with the highest reflectivity while maintaining this performance at high speeds without introducing any distortion to the incident wavefront. Here we demonstrate that these challenges for the MEMS to perform as a dynamic X-ray diffractive optics can be readily met, which unlocks innovative opportunities for their unique use as dynamic X-ray optics. 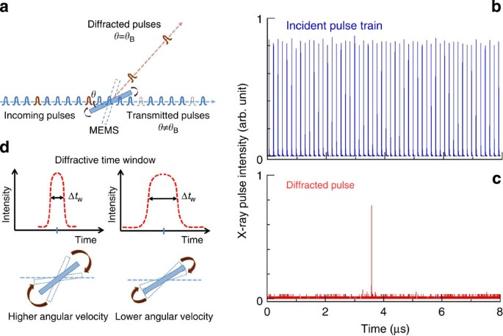Figure 3: MEMS-based dynamic X-ray optics concept. (a) Diffraction of X-ray pulses is realized when the single-crystal MEMS is oriented in the Bragg condition. Otherwise, the X-ray pulses are either absorbed or transmitted. (b) 8-keV X-ray pulses from the APS undulator measured with an avalanche photodiode operated in a charge-integrating mode. The pulses are equally spaced with an interval of 153 ns (6.518 MHz). (c) A single diffracted X-ray pulse selected from the APS pulse train by the oscillating 75-kHz MEMS. (d) The diffractive time window can be varied by changing the angular velocity of the MEMS. Larger amplitude or higher frequency results in a higher angular velocity and hence a smaller time window. Figure 3: MEMS-based dynamic X-ray optics concept. ( a ) Diffraction of X-ray pulses is realized when the single-crystal MEMS is oriented in the Bragg condition. Otherwise, the X-ray pulses are either absorbed or transmitted. ( b ) 8-keV X-ray pulses from the APS undulator measured with an avalanche photodiode operated in a charge-integrating mode. The pulses are equally spaced with an interval of 153 ns (6.518 MHz). ( c ) A single diffracted X-ray pulse selected from the APS pulse train by the oscillating 75-kHz MEMS. ( d ) The diffractive time window can be varied by changing the angular velocity of the MEMS. Larger amplitude or higher frequency results in a higher angular velocity and hence a smaller time window. Full size image If the incident X-ray beam makes an angle θ 0 with the stationary Si crystal, during the oscillation, the time dependence of the incident angle θ ( t ) can be described as θ ( t )= θ 0 + α m cos (2 πf m t ), where α m is the amplitude and f m is the frequency of the MEMS oscillation. The angular velocity of MEMS, ω ( t ), is given by where ω max =2 πf m α m is the maximum angular velocity of the MEMS. The incident X-ray beam is diffracted at the Bragg condition, θ ( t )= θ B , which occurs twice in an oscillation cycle. The value of | ω ( t )/ ω max | is unity at T /4 and 3 T /4 as shown in Fig. 4a , where T =1/ f m is the oscillation period. 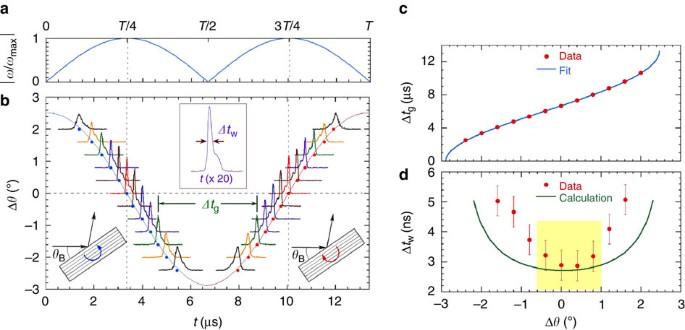Figure 4: MEMS dynamic performance of the MEMS diffractive optics. (a) Normalized angular velocity over one oscillating cycle of MEMS, whereωmax=1.261° μs−1. (b) The experimental data in the time domain where the position and intensity of the 8-keV diffracted X-ray peaks (locally expanded along the time axis by a factor of 20) over the one cycle of the oscillation period are plotted as a function of time and the values of Δθ=θB−θ0. A magnified diffraction profile (at Δθ=0.8°) is shown in the inset. The diffracted peak is narrowest when Δθ=0°. The mirror image of diffraction profiles on the two branches of motion highlights the symmetric rotation of the MEMS. (c) The measured time-gap (Δtg) between the X-ray pulses fits perfectly with equation 2 when the maximum value of the MEMS deflection amplitude is ±2.69°. (d) The width, Δtw, of Si(400) diffraction peak obtained from the time-domain diffraction profiles analysed using the 3-Gaussian model (see text) shown as a function of Δθ. Near Δθ=0° (shaded), the measured values (dots) agree well with calculation using equation 3 (line) with no fitting parameter. Figure 4: MEMS dynamic performance of the MEMS diffractive optics. ( a ) Normalized angular velocity over one oscillating cycle of MEMS, where ω max =1.261° μs −1 . ( b ) The experimental data in the time domain where the position and intensity of the 8-keV diffracted X-ray peaks (locally expanded along the time axis by a factor of 20) over the one cycle of the oscillation period are plotted as a function of time and the values of Δ θ = θ B − θ 0 . A magnified diffraction profile (at Δ θ =0.8°) is shown in the inset. The diffracted peak is narrowest when Δ θ =0°. The mirror image of diffraction profiles on the two branches of motion highlights the symmetric rotation of the MEMS. ( c ) The measured time-gap (Δ t g ) between the X-ray pulses fits perfectly with equation 2 when the maximum value of the MEMS deflection amplitude is ±2.69°. ( d ) The width, Δ t w , of Si(400) diffraction peak obtained from the time-domain diffraction profiles analysed using the 3-Gaussian model (see text) shown as a function of Δ θ . Near Δ θ =0° (shaded), the measured values (dots) agree well with calculation using equation 3 (line) with no fitting parameter. Full size image For a crystal with a rocking curve width Δ θ ( hkl ) (for diffraction plane hkl ), the gap between two consecutive diffraction-windows (in an oscillation cycle), Δ t g , and the width of the diffraction time window, Δ t w , are dependent on the angular offset between the MEMS equilibrium angle, θ 0 at the device resting position and the Bragg angle θ B as Δ θ = θ B − θ 0 (see Supplementary Notes and Supplementary Fig. 3 ), and are given by and We shall emphasize here that Δ θ is not the incident angle, rather it is the parameter that we use to test the dynamic properties of the MEMS when the crystal is rotated away from its equilibrium (or resting position) by the motion of a diffractometer stage. From these equations it can be noted that the smallest width of the diffraction time window, Δ θ ( hkl ) /2 πf m α m , is obtained when Δ θ =0° (when θ 0 = θ B , the position where the resting crystal satisfies the Bragg condition) corresponding to a gap of 1/(2 f m ) between the pulses. The dynamic performance of the MEMS is evaluated from X-ray intensity measurements in the time domain from either a continuous-wave or pulsed X-ray source. In this study we have used the incident X-ray pulse train from the Advanced Photon Source’s standard operating mode in which the pulse-to-pulse separation is 153.4 ns (ref. 24 ). The MEMS device was driven by a 70 V pp actuation signal with frequency 2 f m ( f m =74.671 kHz), resulting in a harmonic oscillation with a nominal amplitude α m of (±)3° and period T of 13.392 μs. During each MEMS oscillation cycle, only the X-ray pulses that satisfy the Bragg condition arriving within the defined Si(400) diffractive time window will be diffracted. This fast pulse modulation capability is shown in Supplementary Data 2 and Supplementary Fig. 4 and is further discussed below. To validate the above concept, time dependence of the 8-keV diffracted X-ray intensities were collected for different offset angle θ 0 . By using the diffracted pulse intensity (similar to that shown in Fig. 3c ), the profile of the diffractive time window is constructed by varying the arrival time of the X-ray pulses with respect to the MEMS driving signal. The measured profile in the time domain is shown in Fig. 4b as a function of the angular offset Δ θ=θ B − θ 0 . For every θ 0 , the Bragg reflection is satisfied only during two short instances in each MEMS oscillation cycle. For clarity, the intensity traces in Fig. 4b are plotted in an expanded time scale by a factor of 20 to make their shapes clearly visible within the oscillation cycle. The observed intensity profiles are mirrored on two branches of the oscillatory cycle, corresponding to the two instances in time when the Bragg condition was met from two rotation directions. Their position on the plot is denoted by the solid dots in the figure. The profiles with similar colours emphasize symmetrical performance of the MEMS in an oscillation cycle. Along the vertical axis, the intensity peaks are offset by the amount of the offset angle Δ θ , ranging from −2.4° to +2.0°, within the nominal oscillation amplitude of the MEMS. The two critical dynamic parameters, Δ t g and Δ t w , can be derived from the position of diffraction peaks, as is illustrated in the figure. The values of Δ t g are plotted in Fig. 4c as a function of the offset angle Δ θ , along with a fit (solid line) using equation 2. The remarkable agreement between the data and the fit allowed accurate and independent determination of the MEMS oscillation amplitude, α m =(2.69±0.01)°, the only fitting parameter in the equation. As reflected in equations 1, 2, 3, this is the most critical parameter necessary to describe all the dynamic properties of the MEMS. The diffraction profiles are normalized and shown in Fig. 4b as a function of the offset angle Δ θ (and the mirror images) retain the features measured in the static rocking curve ( Fig. 2b ). However the width of the Si(400) peak varies with Δ θ (or in time, Δ t w ); in fact, it is inversely proportional to the angular velocity of the MEMS, as expected from equation 3. Of all the peaks in the profiles, the narrowest and highest intensity peaks occur when Δ θ= 0°, at which the MEMS reaches the maximum angular velocity ω max =1.261° μs −1 . The peak width reduces and intensity increases when the angular velocity increases as |Δ θ | decreases ( Fig. 4a,b ). Therefore, the time-domain diffraction profiles can be analysed with confidence using the same three-Gaussian model to extract the width Δ t w of the most prominent Si(400) diffraction peak. The values of Δ t w are shown as a function of Δ θ in Fig. 4d , along with calculated values (solid line) using equation 3 with no adjustable parameters. Within experimental error, the data are adequately accounted for at Δ θ =0° by equation 3, without introducing additional strain-related broadening of the rocking curve, demonstrating negligible dynamic distortion of the MEMS at the X-ray Bragg diffraction angle. Away from this angle, the measured value of Δ t w departs rapidly from that predicted by equation 3, suggesting that the additional broadening of Δ θ (400) stems from a growing amount of strain introduced by dynamic deformation. The dynamic deformation is also evident in Supplementary Data 3 and Supplementary Fig. 5 measured by dynamic optical profilometry. Supplementary Fig. 5a illustrates the surface profile of the mirror at the equilibrium position, where the averaged bending angle is minimal, especially the centre part of the crystal, perfectly supporting the X-ray measurement shown in Fig. 4d . To highlight the narrowest diffractive time window achieved with the MEMS optic, the measured dynamic diffraction profile at Δ θ =0° is shown in detail in Fig. 5 , along with the fit introduced in Fig. 2b , but in the time domain. The resulting Δ t w corresponding to the prominent Si(400) peak is 2.8±0.4 ns. This is in excellent agreement with the value of 2.8 ns obtained from equation 3 using experimentally measured values of Δ θ (400) =0.0034°, α m =2.69° and f m =74.671 kHz. We should emphasize here that this minimal diffractive time window coincides with the angular range (of about a degree, highlighted in Fig. 4d ) where the MEMS oscillation does not cause any dynamic distortion in the Si crystal, providing the opportunity of designing ultrafast but perfect crystal optics. Even at large amplitude oscillations at 75 kHz, utilization of the Bragg condition at the equilibrium positions of the oscillation cycle allows the crystal to maintain a perfect angular-temporal correlation, a characteristic necessary to use X-ray diffractive optics in temporal studies. Parenthetically we note that for one of the many capabilities possible, specifically the function of X-ray pulse selection has been attempted by non-MEMS-based methods with which the time window and repetition rate have been limited by the mechanical strength of the materials and peripheral velocity of the rotating element. Significant improvement of both the performance parameters simultaneously in a single device would be difficult and hence had never been demonstrated. This was possible by miniaturizing the device to the realm of MEMS dimensions where scaling allows for the orders of improvement in both time window and repetition rate. 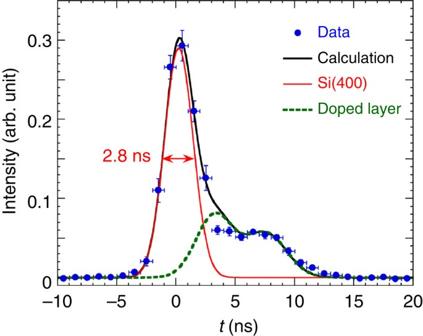Figure 5: The X-ray diffractive time window achieved with 75 kHz MEMS-based diffractive optics. The measured dynamic diffraction profile (dots) at Δθ=0 is fitted with 3-Gaussians (lines). The green curve reflects the peaks associated with a dopant layer identical to those observed in the static diffraction profile. This extra feature will not be present when future MEMS fabrication processes eliminate the inclusion of the dopant layer. The resulting Δtwfor the prominent Si(400) peak is 2.8±0.4 ns in agreement with that obtained from equation 3 using experimentally obtained values of Δθ(400)=0.0034°,αm=2.69° andfm=74.671 kHz. Figure 5: The X-ray diffractive time window achieved with 75 kHz MEMS-based diffractive optics. The measured dynamic diffraction profile (dots) at Δ θ =0 is fitted with 3-Gaussians (lines). The green curve reflects the peaks associated with a dopant layer identical to those observed in the static diffraction profile. This extra feature will not be present when future MEMS fabrication processes eliminate the inclusion of the dopant layer. The resulting Δ t w for the prominent Si(400) peak is 2.8±0.4 ns in agreement with that obtained from equation 3 using experimentally obtained values of Δ θ (400) =0.0034°, α m =2.69° and f m =74.671 kHz. Full size image Our results demonstrate the potential for MEMS technology in the X-ray wavelength range to control the X-ray beam and pulse train from an X-ray source. The current device capability opens many new avenues for the use of MEMS to manipulate and control the spatial, temporal and spectral properties of X-rays similar to the functions demonstrated in the optical wavelength range. Single or an array of the MEMS elements can be used to perform fast scanning of X-ray beams and to manipulate X-ray wave fronts with adaptive controls such as in focusing applications. The MEMS X-ray optics can disperse a well-tailored narrow bandwidth pink X-ray beam by maintaining a one-to-one spatiotemporal correlation with the X-ray energy. This would provide unique opportunities to perform a new class of experiments such as fast time-domain X-ray spectroscopy even with densely filled electron bunches [13] . As shown in Fig. 4d , from Δ θ =−0.5 to +1° (shaded), where minimal dynamic distortion of the mirror is observed, this device can be used as a dynamic (μs) monochromator or spectrometer. With this 1.5° of minimal-distortion range, this device should be capable of dispersing X-rays with a bandwidth of <2% and very high energy resolution (<1 eV) for a densely spaced pulse interval in photon-energy domain ( ∼ 1 eV), suitable for near-edge spectroscopy experiments on microsecond time scales. Using its dynamic diffractive capabilities, the present MEMS can readily be used to select an X-ray pulse or a stream of pulses, with a separation of over 2.8 ns and 150 kHz at any hard X-ray storage ring with dense electron bunch filling patterns. This accounts for most of the present and future-generation sources worldwide. In addition, the X-ray fluence from this optic will be enhanced when applied to the ultra-small beam dimensions obtainable from the new generation of storage-ring sources with sub-nm-rad emittance [25] . The sources will provide much smaller and collimated X-ray beam after focusing and hence smaller (even 10-s μm sized) mirrors can be utilized. With reduced inertia and increased flexure rigidity, faster MEMS can be achievable to significantly increase the performance of the X-ray MEMS optics. Other applications include those that are currently accomplished by bulk X-ray optics such as X-ray phase retarders [26] and beam choppers for nuclear resonance scattering [27] . Another interesting new capability would be to multiplex the X-ray pulses between multiple time-domain experiments at a synchrotron radiation or a high-repetition rate x-ray free electron laser (XFEL) source. Future applications of MEMS X-ray optics hinge on their performance with increased speed (operating at large amplitude in MHz range), small jitter ( ∼ ps), temperature stability and reliability for long-term operation. Fortunately, this is a well evaluated and proven area in photonics applications and can meet their immediate and the future use in X-ray applications discussed below. The four control parameters for MEMS operation at Δ θ =0, namely θ B , Δ θ ( hkl ) , α m , and f m , (equations 1, 2, 3) allow for unprecedented capabilities. They include: (a) the investigation of dynamic processes in a broad range of X-ray energies from ∼ 4 to 50 keV by choosing an appropriate θ B , (b) wafer-scale fabrication of MEMS making it economical to create a scalable catalogue of devices covering a broad range of operation frequencies and ( c ) the values of angular amplitude α m can be varied by orders of magnitude either by varying the applied excitation voltage on MEMS [28] or by varying the ambient pressure in which the device operates [29] , [30] . This would provide flexible diffraction time windows to probe time scales at many MHz rates. MEMS operation with larger values of α m and f m will allow narrower time windows than the few nanoseconds reported here. Ultimately there is a potential to slice the X-ray pulses from a storage-ring synchrotron radiation source by several orders of magnitude to about few picoseconds. How to cite this article: Mukhopadhyay, D. et al. X-ray photonic microsystems for the manipulation of synchrotron light. Nat. Commun. 6:7057 doi: 10.1038/ncomms8057 (2015).